Ancestry of motor innervation to pectoral fin and forelimb Motor innervation to the tetrapod forelimb and fish pectoral fin is assumed to share a conserved spinal cord origin, despite major structural and functional innovations of the appendage during the vertebrate water-to-land transition. In this paper, we present anatomical and embryological evidence showing that pectoral motoneurons also originate in the hindbrain among ray-finned fish. New and previous data for lobe-finned fish, a group that includes tetrapods, and more basal cartilaginous fish showed pectoral innervation that was consistent with a hindbrain-spinal origin of motoneurons. Together, these findings support a hindbrain–spinal phenotype as the ancestral vertebrate condition that originated as a postural adaptation for pectoral control of head orientation. A phylogenetic analysis indicated that Hox gene modules were shared in fish and tetrapod pectoral systems. We propose that evolutionary shifts in Hox gene expression along the body axis provided a transcriptional mechanism allowing eventual decoupling of pectoral motoneurons from the hindbrain much like their target appendage gained independence from the head. Behavioural innovations associated with vertebrate locomotion have depended on functional transformations of the anterior paired appendages. These range from the pectoral fin's role in hydrodynamic mechanisms of balance and swimming to the forelimb's contribution to weight-bearing locomotion [1] . Although the ancestry of these appendages has received much attention [2] , [3] , the evolutionary origin of the corresponding motor circuitry remains largely unexplored. The spinal cord position of tetrapod forelimb circuitry is often presented as the ancestral condition of vertebrates and is presumed to be the location for the corresponding pectoral circuit in bony fish [4] , [5] , [6] , [7] . However, analyses of fish pectoral nerves suggest an alternative organization. Among both main clades of bony vertebrates, sarcopterygian (lobe-finned) and actinopterygian (ray-finned) fish [8] , adult pectoral fins are innervated by spinal nerves, as well as by nerves that exit the posterior, occipital region of the skull [9] , [10] , [11] , [12] . This innervation pattern suggests that pectoral fin motoneurons might originate from both the brain and spinal cord instead of from just the spinal cord. However, nerve trajectory alone cannot be used to identify the ancestral pattern of motor innervation to pectoral appendages because fusion of anterior vertebrae with the occiput during growth can substantially modify the occipital skull [13] . To directly test the hypothesis that pectoral motoneurons have evolutionary and developmental origins from both the hindbrain and spinal cord, we mapped their location in the developing neuroepithelium of actinopterygian fish. Actinopterygians were the main focus of our investigation because, unlike sarcopterygians, the embryos of several species were readily available for the comparative anatomical and molecular analyses essential to determining the ancestry of pectoral neurons and innervation. We included a basal actinopterygian, the acipenseriform Polydon spathula (paddlefish), and several species from the more derived, species-rich group of teleosts [8] . The teleosts chosen were five key study species from three distantly related groups, widely investigated at molecular, neural and behavioural levels of analysis [14] : cypriniforms (zebrafish Danio rerio , goldfish Carassius auratus ), salmoniforms (salmon Salmo salar , trout Salvelinus fontinalis ) and batrachoidiforms (midshipman Porichthys notatus ). Zebrafish included a hoxb4a enhancer trap line [15] expressing a genetic marker demarcating the hindbrain–spinal cord boundary [16] . Using this comparative developmental strategy, we precisely aligned the axial position of developing pectoral motoneurons with other brain nuclei, myotomes and peripheral nerves. We demonstrate that pectoral motoneurons exhibit a conserved pattern of dual origin in both the hindbrain and spinal cord with no migration throughout development. Together with new and previous evidence for occipital and spinal innervation of pectoral fins in sarcopterygian (lungfishes and coelacanth) and more basal cartilaginous (chimaera) fish, the results indicate that this pattern of pectoral innervation is the primitive condition for jawed vertebrates. Pectoral motor control centred at a hindbrain–spinal location was likely a novel adaptation for head orientation and swimming manoeuvres via the occipital–pectoral skeletal connection in primitive fish, including those that gave rise to tetrapods. Location of embryonic pectoral motoneurons The pectoral fin is innervated by a plexus of nerves, members of which are designated as either occipital (Oc) or spinal (Sp) depending on the location of their roots relative to the cranio–vertebral interface [9] , [10] , [11] , [12] . In all four actinopterygians studied, including midshipman ( Fig. 1a ) and zebrafish ( Fig. 1b ), the anterior most pectoral nerve emerged from the skull through an occipital foramen or the foramen magnum (for example, Fig. 1c,d ; Supplementary Figs S1 , S2 ). Although the innervation pattern was grossly conserved, the substantial modifications in the occipital skull produced by its fusion with parts of anterior vertebrae [13] precluded a conclusive comparison between species. We found, however, that alignment of the fin bud, myotomes and neuroepithelium was strikingly similar at early fin bud stages of development across all four species ( Fig. 1e ; Supplementary Fig. S3 ). This finding allowed us to study pectoral innervation at comparable embryonic stages across taxa, independent of species-specific skeletal modifications during subsequent growth. 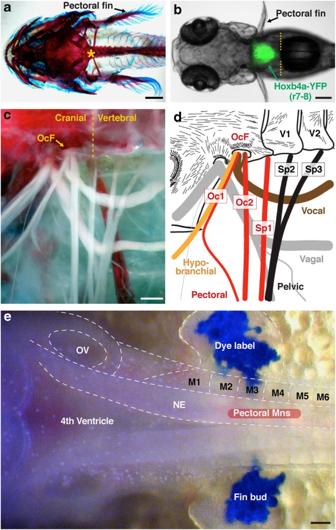Figure 1: Occipital region in actinopterygian fish. (a) Cranio–vertebral junction (asterisk) in a juvenile midshipman stained with alcian blue and alizarin red. (b) Hindbrain–spinal cord boundary (yellow hatching) demarcated in the zebrafishhoxb4aenhancer trap line. (c) Pectoral fin innervation in juvenile midshipman. (d) Schematic drawing ofcshowing occipital nerves (Oc, red, orange and brown ind) exiting through occipital foramen (OcF) located anterior to the cranio–vertebral junction, and spinal nerves (Sp, black ind) exiting through vertebrae (V). (e) Embryonic alignment of caudal hindbrain, fourth ventricle, otic vesicle (OV) and myotomes (M) (includes blue lipophilic dye injection in fin buds; midshipman fish). The location of pectoral motoneurons is also indicated. NE, neuroepithelium. Images are dorsal (a,b,e) and ventral (c,d) views with anterior to the left. Scale bars are 1 cm (a), 200 μm (b), 500 μm (c,d) and 100 μm (e). Figure 1: Occipital region in actinopterygian fish. ( a ) Cranio–vertebral junction (asterisk) in a juvenile midshipman stained with alcian blue and alizarin red. ( b ) Hindbrain–spinal cord boundary (yellow hatching) demarcated in the zebrafish hoxb4a enhancer trap line. ( c ) Pectoral fin innervation in juvenile midshipman. ( d ) Schematic drawing of c showing occipital nerves (Oc, red, orange and brown in d ) exiting through occipital foramen (OcF) located anterior to the cranio–vertebral junction, and spinal nerves (Sp, black in d ) exiting through vertebrae (V). ( e ) Embryonic alignment of caudal hindbrain, fourth ventricle, otic vesicle (OV) and myotomes (M) (includes blue lipophilic dye injection in fin buds; midshipman fish). The location of pectoral motoneurons is also indicated. NE, neuroepithelium. Images are dorsal ( a , b , e ) and ventral ( c , d ) views with anterior to the left. Scale bars are 1 cm ( a ), 200 μm ( b ), 500 μm ( c , d ) and 100 μm ( e ). Full size image Pectoral motoneurons were visualized by injecting a saturated solution of fluorescent lipophilic dye (DiD) into the fin bud that was incorporated into individual axons and diffused along the membrane to label the cell body. Subsequent confocal imaging revealed a consistent dual hindbrain–spinal origin of pectoral motoneurons in actinopterygians. Embryonic pectoral motor nuclei always extended as a column between myotomes (M) 2–3 and 5–6, with separate nerve roots projecting through each successive myotome, starting invariantly with M2 ( Fig. 2a–d ). Location of the embryonic cranio–vertebral [17] and hindbrain–spinal [16] junctions between M3 and 4 showed the pectoral column to be in both the caudal hindbrain and rostral spinal cord with the fin innervated by Oc and Sp nerves ( Fig. 2a–d ; Supplementary Movie 1 ). Taken together, our results indicate that basal and derived actinopterygians share a conserved blueprint, with a hindbrain–spinal pectoral motor nucleus innervating the fin via both Oc and Sp nerves. 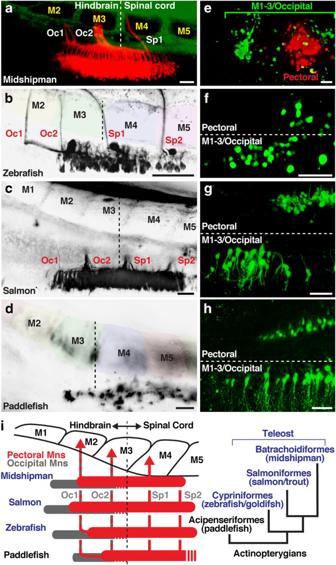Figure 2: Embryonic alignment of pectoral and occipital motoneurons with nerves and myotomes in basal and derived actinopterygians. (a–d) Location of pectoral motoneurons and nerves in actinopterygians revealed by lipophilic dye labelling from fin buds. The pectoral motor column began at the level of myotomes (M) 2–3 in all species studied (vertical hatching marks hindbrain–spinal boundary; also seeFigure 1b,e). (e–h) Double labelling with fluorescent dextrans from fin buds and M1–3 showed that the occipital motor column began one myotomal segment anterior to pectoral motoneurons. Horizontal hatching marks midline inf–h. (i) Alignment of myotomes, nerves and motoneurons (pectoral/red and occipital/grey) with phylogenetic relationships of actinopterygians studied here (right). Paddlefish innervation pattern was deduced from juvenile gross anatomy (Supplementary Fig. S1,S2) as individual roots were not clearly visualized using retrograde labelling. All images are dorsal views with anterior to the left. Scale bars are 50 μm. Specimen stages:a(10 days postfertilization (dpf)/~5.5 mm),b(2 dpf/~3 mm),c(100 dpf/~10 mm),d(9 dpf/~13 mm),e(18 dpf/~11 mm),f(4 dpf/~4 mm),g(115 dpf/~12 mm),h(11 dpf/~16 mm). Figure 2: Embryonic alignment of pectoral and occipital motoneurons with nerves and myotomes in basal and derived actinopterygians. ( a – d ) Location of pectoral motoneurons and nerves in actinopterygians revealed by lipophilic dye labelling from fin buds. The pectoral motor column began at the level of myotomes (M) 2–3 in all species studied (vertical hatching marks hindbrain–spinal boundary; also see Figure 1b,e ). ( e – h ) Double labelling with fluorescent dextrans from fin buds and M1–3 showed that the occipital motor column began one myotomal segment anterior to pectoral motoneurons. Horizontal hatching marks midline in f – h . ( i ) Alignment of myotomes, nerves and motoneurons (pectoral/red and occipital/grey) with phylogenetic relationships of actinopterygians studied here (right). Paddlefish innervation pattern was deduced from juvenile gross anatomy ( Supplementary Fig. S1 , S2 ) as individual roots were not clearly visualized using retrograde labelling. All images are dorsal views with anterior to the left. Scale bars are 50 μm. Specimen stages: a (10 days postfertilization (dpf)/~5.5 mm), b (2 dpf/~3 mm), c (100 dpf/~10 mm), d (9 dpf/~13 mm), e (18 dpf/~11 mm), f (4 dpf/~4 mm), g (115 dpf/~12 mm), h (11 dpf/~16 mm). Full size image Alignment with central and peripheral landmarks Precise, three-dimensional neuronal maps were obtained by aligning hindbrain nuclei with myotomes and peripheral nerves, complemented in transgenic zebrafish lines by genetic markers that label motoneuronal pools and demarcate the hindbrain–spinal boundary between M3 and 4. We first identified all hindbrain motoneurons exiting via Oc nerves by fluorescent labelling from the three most anterior myotomes, M1–3. In all cases, labelled occipital motoneurons formed a ventral column that began about one myotomal segment anterior to the pectoral column ( Fig. 2e–h ). The occipital column included all posterior hindbrain neurons projecting through Oc roots innervating pectoral fin, hypobranchial and axial (M1–3) muscles [10] (summarized in Figure 2i ). This overlapping occipital pectoral motoneuronal pattern further supported a generic blueprint of hindbrain–spinal pectoral innervation in actinopterygians. We next aligned the pectoral motoneurons with other central nuclei using transgenic zebrafish lines. In the hoxb4a enhancer trap background ( Figs 1b and 3a ), a gata-2 promotor-driven YFP was inserted 3-kb downstream of the endogenous hoxb4a gene [15] . Many neurons from rhombomeres (r) 7–8 are genetically labelled with YFP, reflecting the presence of hoxb4a enhancer activity [16] ( Fig. 3a,b ). The retrogradely labelled pectoral motor column was located in posterior r8 and extended into the adjacent spinal cord ( Fig. 3c ). Notably, the retrogradely labelled occipital motor column extended further rostral than pectoral motoneurons into the middle of r8 ( Fig. 3d ). Double labelling from the fin and cerebellum in an islet1 -GFP transgenic background [18] showed the hindbrain pectoral motoneurons to be located immediately caudal to precerebellar neurons (inferior olive/IO and area II/AII) in the middle of r8 [16] ( Fig. 3e–g ; Supplementary Movie 2 ). A similar alignment of precerebellar and pectoral neurons in other teleosts studied (midshipman, trout and goldfish; Supplementary Fig. S4 ) strongly supported a common hindbrain neuronal map for actinopterygians. Occipital and pectoral motoneurons formed a single column (Oc/Pec) that was directly ventral to the posterior half of the vagal (X) motor nucleus in the caudal hindbrain and extended into the anterior spinal cord ( Fig. 3h ; also see Fig. 2e–h ). 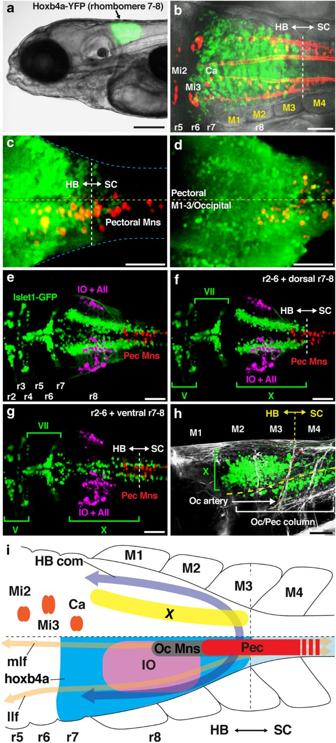Figure 3: Embryonic alignment of precerebellar, pectoral and other hindbrain neurons in transgenic zebrafish. (a) Rhombomere (r) 7–8 YFP expression inhoxb4aenhancer trap line. (b) Reticular (labelled from the spinal cord; red) and YFP (green) neurons showed hindbrain–spinal cord boundary between myotomes (M) 3–4. (c) Half of the pectoral column (labelled from fin bud; red) was within the hindbrain. (d) Occipital motor column (labelled from M1–3/occipital) extended to mid r8, one segment rostral to pectoral motoneurons. (e–g) Dorsal composites (e) and selected confocal planes (f,g) of pectoral (labelled from fin buds; red), inferior olive (IO) and Area II (AII) (labelled from the cerebellum; magenta) neurons inislet-GFP background (green), showing the relative position of pectoral motoneurons with major neuronal subgroups. GFP in this line is expressed in all hindbrain motoneurons, except abducens and pectoral. (h) Vagal (X) and more ventral occipital (Oc) motor columns that extended from spinal cord into the hindbrain (also seef,g). (i) Alignment of pectoral motoneurons (Pec) with other neuronal and anatomical landmarks. Pectoral motoneurons in zebrafish were located across the hindbrain–spinal cord boundary at the level of M3–5 (seeFigure 2). Hindbrain motoneurons are located immediately caudal to the inferior olive, below the vagal nucleus (X) and hindbrain commissure (HB com). They are part of the occipital motor column (Oc Mns) at the level of two fibre tracts, the medial longitudinal fasciculus (mlf) and the lateral longitudinal fasciculus (llf). Other abbreviations: Mi2, Mi3 and Ca, reticulospinal neurons53. Images are dorsal (b,c,e–g,i), ventral (d) and lateral (a,h) views with anterior to the left. Scale bars are 200 μm (a), 50 μm (b–h). Specimen stages:a,c,d(4 dpf),b(2 dpf),e–h(5 dpf). Neuronal mapping with genetically and retrogradely labelled neurons thus showed pectoral motoneurons distributed across the hindbrain–spinal cord boundary and precisely positioned them with respect to other hindbrain subgroups (summarized in Figure 3i ). Figure 3: Embryonic alignment of precerebellar, pectoral and other hindbrain neurons in transgenic zebrafish. ( a ) Rhombomere (r) 7–8 YFP expression in hoxb4a enhancer trap line. ( b ) Reticular (labelled from the spinal cord; red) and YFP (green) neurons showed hindbrain–spinal cord boundary between myotomes (M) 3–4. ( c ) Half of the pectoral column (labelled from fin bud; red) was within the hindbrain. ( d ) Occipital motor column (labelled from M1–3/occipital) extended to mid r8, one segment rostral to pectoral motoneurons. ( e – g ) Dorsal composites ( e ) and selected confocal planes ( f , g ) of pectoral (labelled from fin buds; red), inferior olive (IO) and Area II (AII) (labelled from the cerebellum; magenta) neurons in islet -GFP background (green), showing the relative position of pectoral motoneurons with major neuronal subgroups. GFP in this line is expressed in all hindbrain motoneurons, except abducens and pectoral. ( h ) Vagal (X) and more ventral occipital (Oc) motor columns that extended from spinal cord into the hindbrain (also see f , g ). ( i ) Alignment of pectoral motoneurons (Pec) with other neuronal and anatomical landmarks. Pectoral motoneurons in zebrafish were located across the hindbrain–spinal cord boundary at the level of M3–5 (see Figure 2 ). Hindbrain motoneurons are located immediately caudal to the inferior olive, below the vagal nucleus (X) and hindbrain commissure (HB com). They are part of the occipital motor column (Oc Mns) at the level of two fibre tracts, the medial longitudinal fasciculus (mlf) and the lateral longitudinal fasciculus (llf). Other abbreviations: Mi2, Mi3 and Ca, reticulospinal neurons [53] . Images are dorsal ( b , c , e – g , i ), ventral ( d ) and lateral ( a , h ) views with anterior to the left. Scale bars are 200 μm ( a ), 50 μm ( b – h ). Specimen stages: a , c , d (4 dpf), b (2 dpf), e – h (5 dpf). Full size image In situ origination of hindbrain pectoral motoneurons The dual hindbrain–spinal origin of pectoral motoneurons was explicitly demonstrated using the photoconvertible protein kaede [19] to trace the fate of the neuroepithelium in the hindbrain and anterior spinal cord, starting from early neurogenesis ( Fig. 4a–e ; Supplementary Movie 3 ). Kaede in both neuroepithelium and somites at the level of somites 4–5 was photoconverted from green to red at 12 h postfertilization (hpf; early neural keel stage [20] ; Fig. 4a,b ) or at 18 hpf (neural rod stage [20] ). Subsequent confocal analysis at 2 days postfertilization (dpf) showed that red kaede-labelled neurons remained at the level of M4–5 ( Fig. 4c ). Neurons located maximally 2–3 cell diameters away from the photoconverted area were occasionally observed (arrows, Fig. 4c ). Retrograde labelling showed that pectoral motoneurons in the hindbrain at the level of M3 ( Fig. 4c,d ) did not contain the red converted version of kaede, unlike those in the anterior spinal cord ( Fig. 4c,e ). Pectoral motoneurons exhibited minimal, if any, anterior–posterior migration, regardless of whether the photo-conversion was performed either at 12 hpf ( n = 11) or 18 hpf ( n = 10), or at the level of M3–4 ( n = 2), M4–5 ( n = 21) or M5–6 ( n = 7). 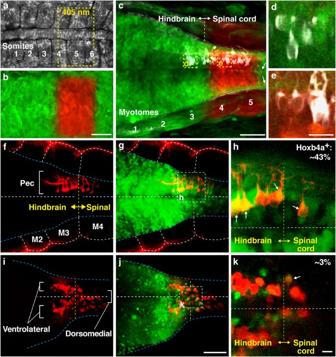Figure 4: Origin and maintenance of pectoral motoneurons across the hindbrain–spinal cord boundary. (a) Future hindbrain–spinal cord region in a 12 h postfertilization (hpf) embryo showing somites 1–6. (b) Transiently expressed kaede protein was photoconverted from green to red at the level of somites 4–5. Yellow dashed line in (a) marks the area of photoconversion using a laser of 405 nm. (c) The same embryo at 2 days postfertilization (dpf) showed minimal, if any, anterior–posterior migration, with labelled neurons remaining tightly clustered at the level of myotomes (M) 4–5. Arrows point to neurons that were displaced 2–3 cell diameters posteriorly. (d,e) High magnification single plane images showed photoconverted kaede to be absent in pectoral motoneurons (white) at the level of M3 (d), but present in those at the level of M4 (e). (f–k) Ontogeny of pectoral motoneurons. At 2 dpf, pectoral motoneurons were labelled with lipophilic dye from fin bud (red) and appeared as a single column at the level of M3–4 (f) where they overlapped with thehoxb4a-YFP (green) expression domain (g, shown at a higher magnification inh). At 20 dpf, pectoral motoneurons increased in number and developed into paired ventrolateral and dorsomedial columns (i). The motoneurons remained across the hindbrain–spinal cord boundary (yellow dashed line inj) demarcated by YFP expression (shown at a higher magnification ink) and exhibited a progressive downregulation ofhoxb4aactivity16(arrows;h,k). Images are dorsal (a–h) and ventral (i–k) views with anterior to the left. Scale bars are 50 μm (a–c,f,g,i,j) and 10 μm (d,e,h,k). Specimen stages:a,b(12 hpf),c–h(2 dpf) andi–k(20 dpf). Figure 4: Origin and maintenance of pectoral motoneurons across the hindbrain–spinal cord boundary. ( a ) Future hindbrain–spinal cord region in a 12 h postfertilization (hpf) embryo showing somites 1–6. ( b ) Transiently expressed kaede protein was photoconverted from green to red at the level of somites 4–5. Yellow dashed line in ( a ) marks the area of photoconversion using a laser of 405 nm. ( c ) The same embryo at 2 days postfertilization (dpf) showed minimal, if any, anterior–posterior migration, with labelled neurons remaining tightly clustered at the level of myotomes (M) 4–5. Arrows point to neurons that were displaced 2–3 cell diameters posteriorly. ( d , e ) High magnification single plane images showed photoconverted kaede to be absent in pectoral motoneurons (white) at the level of M3 ( d ), but present in those at the level of M4 ( e ). ( f – k ) Ontogeny of pectoral motoneurons. At 2 dpf, pectoral motoneurons were labelled with lipophilic dye from fin bud (red) and appeared as a single column at the level of M3–4 ( f ) where they overlapped with the hoxb4a -YFP (green) expression domain ( g , shown at a higher magnification in h ). At 20 dpf, pectoral motoneurons increased in number and developed into paired ventrolateral and dorsomedial columns ( i ). The motoneurons remained across the hindbrain–spinal cord boundary (yellow dashed line in j ) demarcated by YFP expression (shown at a higher magnification in k ) and exhibited a progressive downregulation of hoxb4a activity [16] (arrows; h , k ). Images are dorsal ( a – h ) and ventral ( i – k ) views with anterior to the left. Scale bars are 50 μm ( a – c , f , g , i , j ) and 10 μm ( d , e , h , k ). Specimen stages: a , b (12 hpf), c – h (2 dpf) and i – k (20 dpf). Full size image Ontogeny of pectoral motoneurons The location of pectoral motoneurons was further examined throughout early development by alignment in the hoxb4a enhancer trap background ( Fig. 4f–k ). During 2–20 dpf, when both pectoral musculature and innervation attain an adult configuration [21] , [22] , pectoral motoneurons increased in number in both hindbrain and spinal cord, splitting from a single motor pool into ventrolateral and dorsomedial columns ( Fig. 4f,i ). Their relative position to the hoxb4a -YFP domain indicated that pectoral motoneurons originated from, and were maintained, across the hindbrain–spinal cord boundary ( Fig. 4g,h,j,k ). On the basis of axonal trajectory, there was no evidence for pectoral motoneuron migration along the anterior–posterior axis ( Fig. 4i–k ). Taken together with the kaede experiments, these data demonstrated that pectoral motoneurons did not exhibit any longitudinal migration from early neurogenesis through later development, similar to postmitotic spinal motoneurons in tetrapods [23] . Thus, pectoral motoneurons originated and remained across the hindbrain–spinal boundary in actinopterygian fish [23] . Pectoral innervation in Chondrichthyes and Dipnoi To facilitate comparisons with more readily available juvenile/adult sarcopterygian and the even more primitive cartilaginous fish/Chondrichthyes [8] , we investigated pectoral innervation in two lungfish/Dipnoi species ( Protopterus dolloi and Lepidosiren paradoxa ) and ratfish/Chimaeriformes ( Hydrolagus colliei ). Ratfish had four Oc nerves (Oc1–4) that originated from the hindbrain as ventral roots directly behind the vagus nerve (X). All four nerve roots immediately combined into one nerve ( Fig. 5a ) that branched into hypobranchial and pectoral nerves at the level of the pectoral girdle (inset, Fig. 5a ). The pectoral nerve immediately joined Sp nerves 1–3 to form a plexus (inset, Fig. 5a ) that innervated the pectoral fin along with 11 separate Sp nerve branches ( Fig. 5a ). Lungfish had three Oc nerves ( Fig. 5b ; Supplementary Fig. S5 ), with the most posterior root (Oc3) emerging from the caudal hindbrain at a level near the end of the fourth ventricle ( Fig. 5b ). The Oc3 dorsal and ventral roots exited via two separate cranial foramina and fused into a single nerve immediately outside the skull ( Supplementary Fig. S5a ). Oc3 later merged with Sp1–3, forming a single pectoral nerve ( Fig. 5 ; Supplementary Fig. S5 ). In summary, cartilaginous and sarcopterygian fish exhibited Oc and Sp innervation of the pectoral fin, similar to actinopterygians, supporting the hypothesis that a dual hindbrain–spinal origin of pectoral motoneurons is an ancestral trait for jawed (cartilaginous and bony) vertebrates (summary, Fig. 6a ). 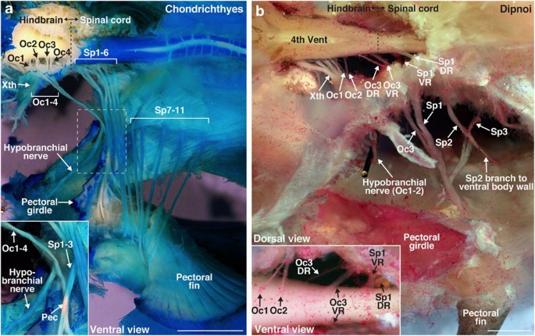Figure 5: Pectoral innervation in Chondricthyes (ratfish) and Dipnoi (lungfish). (a) Pectoral innervation in ratfish (H. colliei) included four occipital (Oc1–4) and 11 spinal nerves (Sp1–11). Inset shows the branching of Oc1–4 contributing to both hypobranchial nerve and the pectoral plexus. (b) Pectoral innervation in spotted African lungfish (P. dolloi) included one occipital (Oc3) and three spinal nerves (Sp1–3). Oc3 dorsal (DR) and ventral (VR) roots emerged at the caudal end of the hindbrain. Inset shows the ventral view of Oc1–3 and Sp1. Scale bars are 5 mm. Figure 5: Pectoral innervation in Chondricthyes (ratfish) and Dipnoi (lungfish). ( a ) Pectoral innervation in ratfish ( H. colliei ) included four occipital (Oc1–4) and 11 spinal nerves (Sp1–11). Inset shows the branching of Oc1–4 contributing to both hypobranchial nerve and the pectoral plexus. ( b ) Pectoral innervation in spotted African lungfish ( P. dolloi ) included one occipital (Oc3) and three spinal nerves (Sp1–3). Oc3 dorsal (DR) and ventral (VR) roots emerged at the caudal end of the hindbrain. Inset shows the ventral view of Oc1–3 and Sp1. Scale bars are 5 mm. 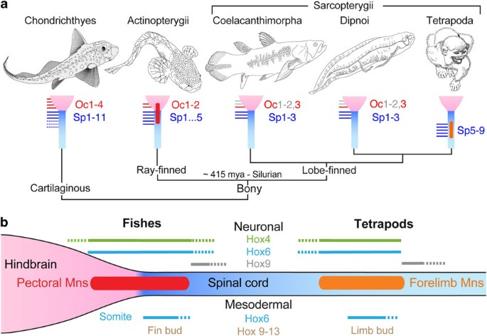Figure 6: Evolution of pectoral innervation. (a) Cladogram of living jawed vertebrates8, with vignettes showing innervation patterns of pectoral appendages. Occipital (pectoral, red; hypobranchial, grey) and spinal (blue) nerves are illustrated schematically. (b) Summary of keyHoxgenes expressed in neuronal (top) and mesodermal (bottom) compartments along the anterior–posterior axis in fish and tetrapods43,46,47,49,51. Full size image Figure 6: Evolution of pectoral innervation. ( a ) Cladogram of living jawed vertebrates [8] , with vignettes showing innervation patterns of pectoral appendages. Occipital (pectoral, red; hypobranchial, grey) and spinal (blue) nerves are illustrated schematically. ( b ) Summary of key Hox genes expressed in neuronal (top) and mesodermal (bottom) compartments along the anterior–posterior axis in fish and tetrapods [43] , [46] , [47] , [49] , [51] . Full size image The conserved pectoral innervation pattern among jawed fish shown here, which consists of motoneurons and nerves originating from both the hindbrain and the spinal cord, differs notably from the spinal-only innervation in tetrapods. Our work in basal and derived actinopterygians supports the hypothesis that a dual hindbrain–spinal origin for pectoral motoneurons in fish evolved into a spinal-only origin for forelimb motoneurons in tetrapods. This proposal is corroborated by new and previous evidence of pectoral innervation from hindbrain/Oc and Sp nerves in lobe-finned and cartilaginous fish, implying that the pectoral motoneuron pool, similar to its target appendage, shifted caudally along the anterior–posterior axis during the fin-to-limb transition [24] . Our embryonic data showed pectoral motoneurons located in the hindbrain of four actinopterygian species ( Figs 2 , 3 , 4 ). Lineage tracing showed that these neurons originated in embryonic sites in both the hindbrain and spinal cord that were maintained throughout ontogeny in zebrafish ( Figs 3 and 4 ). This embryonic blueprint was conserved among basal and derived actinopterygians ( Fig. 2 ) and gave rise to adult innervation consisting of two Oc and various numbers (1–5) of Sp nerves ( Figs 1 and 2 ; Supplementary Figs S1 , S2 ). We conclude that a dual hindbrain–spinal origin is the primitive trait for actinopterygian fish ( Fig. 6a ). Sarcopterygians, the sister group of actinopterygians, also exhibited an occipital-spinal pectoral nerve pattern. As in the living coelacanth/ Latimeria [25] , [26] , pectoral innervation in two species of lungfish/Dipnoi included an Oc nerve (Oc3) that originated from the hindbrain ( Fig. 5 ; Supplementary Fig. S5 ). Similar to actinopterygians, the spinal contribution to pectoral innervation varied among sarcopterygians (11 in Latimeria versus 3 in P. dolloi ). Together with our embryological results, we conclude that a hindbrain contribution to pectoral appendage innervation is the primitive condition for bony fish, including the sarcopterygians that gave rise to tetrapods ( Fig. 6a ). We expanded our analysis to the most basal group of living jawed fish, Chondrichthyes, which include two subclasses, holocephalans such as the ratfish studied here and elasmobranchs (sharks and batoids). Pectoral innervation in ratfish, as in all other species studied here, involved Oc and Sp nerves ( Fig. 5a ). Hindbrain pectoral neurons were also reported in a batoid [27] , unlike the Sp-only innervation reported in sharks [28] , [29] . We propose that Oc/Sp pectoral innervation among actinopterygians, sarcopterygians and members of both subclasses of chondrichthyans (the elasmobranch pattern may be derived) represents the ancestral condition for all jawed vertebrates. The general blueprint of a hindbrain–spinal motor column innervating occipital, hypobranchial and pectoral muscles ( Figs 2i and 3i ) is likely an ancestral feature linked to the original skull-fin musculoskeletal complex in fish ( Fig. 6a ). Fossil cephalaspids (jawless fishes/ostracoderms) exhibited well-developed pectoral fins that likely provided hydrodynamic lift, contributing to head orientation and sharp manoeuvres during swimming [30] . The fins were suggested to be innervated by the most anterior 2–3 ventral roots that emerged directly behind the vagus nerve [31] , [32] , similar to the condition in living jawed fish ( Figs 1 , 5 and 6 ; Supplementary Figs S1 , S2 , S5 ). The endoskeleton of cephalaspid pectoral fins was articulated to the cranium [33] , [34] , analogous to the pectoral–occipital connection in early fossil sarcopterygians and primitive actinopterygians [33] , [35] that share a similar pectoral endoskeletal structure [36] , [37] . The decoupling of this articulation and consequent increase in head mobility during the water-to-land transition, as seen in the fossil sarcopterygian fish Tiktaalik roseae [2] , [38] , may have been the reason for pectoral innervation being dissociated from the hindbrain. Unlike in fish, caudal hindbrain ventral roots in living amphibians contribute to Sp nerves 1–2 that innervate occipital, hypobranchial and hypoglossal muscles. Pectoral innervation typically arises from Sp nerves 3–5, with forelimb motoneurons located in the rostral spinal cord [4] , [5] . These observations in amphibians suggest that pectoral forelimb innervation in early tetrapods may have been shifted only a few segments caudally, relative to the pattern seen in sarcopterygian fish, despite separation of the skull and pectoral girdle [38] , [39] . In amniotes, there are generally six or more cervical vertebrae [40] giving rise to a more elaborated neck structure. The rostral limit of pectoral forelimb innervation varies from Sp nerve 4 in some reptiles and mammals to Sp nerve 22 in long-necked birds [6] , [41] , [42] , [43] , [44] . As lower numbers of cervical vertebrae seem to be primitive for amniotes [40] , it seems that a caudal shift of about 5–6 segments in the location of the pectoral plexus, and therefore the motor nuclei, occurred between sarcopterygian fish and early amniotes ( Fig. 6a ). The absence of forelimb motoneurons in the tetrapod hindbrain can thus be viewed as the neuronal complement to the loss of the occipital–pectoral skeletal connection and the increased independence of head and body motion during the emergence of terrestrial vertebrates [2] , [38] . The repositioning of both pectoral motoneurons and the pectoral girdle along the body axis likely depended, in part, on evolutionary developmental changes in the blueprint of Hox gene expression, which is important for both neuroectoderm and mesoderm patterning along the anterior–posterior axis [45] . The Hox regulatory framework is presumed to have instructed a repositioning of pectoral fin/forelimb in vertebrates [43] . The same mechanism likely positioned the motor column along with appendages at the corresponding axial level ( Fig. 6b ), as exemplified by Hox gene expression in both pectoral [16] and forelimb [46] motoneurons. A comparison of Hox expression data from previous studies [43] , [46] , [47] , [48] , [49] shows that fish and tetrapods share highly similar neuronal and mesodermal Hox codes for 'positioning' [43] and 'patterning' [46] the pectoral appendage and motoneuronal pool ( Fig. 6b ). Thus, the Hox code for both musculoskeletal and neuronal compartments is conserved for the pectoral motor system, despite anatomical differences in location along the anterior–posterior axis. As summarized in Figure 6b , we propose that the posterior shift of the pectoral motor nucleus involved sets of cis -regulatory changes in Hox genes that led to both loss of pectoral-related transcriptional machinery in the tetrapod hindbrain and correlated changes in the occipital, cervical and pectoral appendage peripheries [43] , [46] , [47] , [49] , [50] , [51] . In birds and mammals, Hox6 and Hox9 paralogous groups confer, respectively, cervical and thoracic identity onto the neuroectoderm along the anterior–posterior axis [46] . In zebrafish, similar to birds and mammals, the anterior expression limits of Hox6 / 9 bracket the rostral–caudal extent of the pectoral motoneuron region [48] , [49] ( Fig. 6b ). Therefore, the spatial relationship of Hox6 / 9 and pectoral motoneuron location has essentially been maintained during the caudal repositioning of the forelimb motor column ( Fig. 6b ). Similarly, in the mesoderm, the relative position of Hox6 expression and the axial level of limb/fin bud outgrowth seem to be conserved during pectoral appendage relocation between fish and tetrapods [43] ( Fig. 6b ). Subsequent patterning of pectoral appendages also involves Hox9–13 triphasic expression in both zebrafish [47] and tetrapods [51] . After early regionalization of the neuroectoderm, Hox3–8 paralogous groups define forelimb motoneuron pools in birds and mammals [46] . The same set of Hox genes is expressed in the hindbrain–spinal region that gives rise to pectoral motoneurons in zebrafish [48] , [49] . Hence, we predict the presence of Hox3–8 in pectoral motoneurons, similar to their tetrapod counterparts, although only Hox4 has been directly demonstrated so far [16] ( Fig. 6b ). Conserved expression patterns in neuroectoderm, mesoderm and pectoral appendages are together suggestive of an ancestral neuronal/mesodermal Hox network linking motoneurons in both the hindbrain and spinal cord with the pectoral periphery ( Fig. 6b ). The evolutionary plasticity afforded by this Hox network provided a basis for further innovations in neural circuitry controlling forelimb functions essential to novel mechanisms of locomotion and feeding in tetrapods [2] , [38] . Animals and specimens Paddlefish were obtained from Osage Catfisheries (Osage Beach), salmon embryos from Grand Lake Stream Fish Hatchery, salmon juveniles and brook trout embryos from C Kraft and D Josephson (Department of Natural Resources, Cornell University, Ithaca, NY), goldfish from Hunting Greek Fisheries, midshipman from M Marchaterre (Department of Neurobiology and Behavior, Cornell University, Ithaca, NY), fixed specimens of ratfish from J Sisneros (Department of Psychology, University of Washington, Seattle, WA, USA) and South American and South African lungfishes from Tropical Fish Distributors. Animal handling and experimental procedures were approved by the Institutional Animal Care and Use Committee of New York University School of Medicine (New York, NY, USA), Cornell University (Ithaca, NY, USA) and Marine Biological Laboratory (Woods Hole, MA, USA). Fixation and staining for gross anatomy Juveniles/adults were killed by an overdose of ethyl 3-aminobenzoate methanesulphonate (MS 222, Sigma), fixed by 4% paraformaldehyde perfusion and then stained sequentially with alcian blue and alizarin red before dissection [52] . For some paddlefish, nerves were stained briefly with 2% osmium tetroxide solution after fixation. Retrograde labelling Embryos and larvae were anaesthetized with 0.02% MS 222 and immobilized in 2% low-gelling agarose for imaging [16] . For retrograde labelling in early embryos, 50–100 nl of saturated mixture of the lipophilic dye DiD (Invitrogen) in 50% vegetable oil/50% dimethylsulphoxide was pressure injected into the fin bud at 40 psi. As lipophilic dye works very poorly in live specimens later in development, pectoral motoneurons in larvae were labelled by injecting 200–300 nl of Alexa Fluor 647 dextran (3% in 0.2 KCl with 0.1% Triton X-100) into the fin musculature. Double labelling of either Oc or precerebellar neurons was achieved by additional dye injection into, respectively, M1–3 (~200 nl of either Alexa Flour 488 or 647 dextran; 3% in 0.2 KCl with 0.1% Triton X-100) or the cerebellum (~50 nl of either Alexa Fluor 488 or 594 dextran; 3% in 0.2 KCl with 0.1% Triton X-100) [16] . Kaede lineage tracing Lineage tracing experiments were conducted by injecting 500 pg of mRNA encoding the photoconvertable protein kaede into single-cell-stage zebrafish embryos [19] . Neuroepithelium and somites at the level of somites 4–5 were scanned by a laser of 405 nm on a confocal microscope at either 12 or 18 hpf, which induced green-to-red photoconversion of cytosolic kaede protein. Lineage of cells containing converted kaede was examined using a confocal microscope at 2 dpf. Confocal images were obtained using a Zeiss 510 system and processed using ImageJ (NIH) and Photoshop (Adobe). How to cite this article: Ma, L.-H. et al . Ancestry of motor innervation to pectoral fin and forelimb. Nat. Commun. 1:49 doi: 10.1038/ncomms1045 (2010).